Revealing the fast atomic motion of network glasses Still very little is known on the relaxation dynamics of glasses at the microscopic level due to the lack of experiments and theories. It is commonly believed that glasses are in a dynamical arrested state, with relaxation times too large to be observed on human time scales. Here we provide the experimental evidence that glasses display fast atomic rearrangements within a few minutes, even in the deep glassy state. Following the evolution of the structural relaxation in a sodium silicate glass, we find that this fast dynamics is accompanied by the absence of any detectable aging, suggesting a decoupling of the relaxation time and the viscosity in the glass. The relaxation time is strongly affected by the network structure with a marked increase at the mesoscopic scale associated with the ion-conducting pathways. Our results modify the conception of the glassy state and asks for a new microscopic theory. Understanding the relaxation dynamics of glasses is still considered as one of the most challenging issues in solid state physics [1] , [2] . On approaching the glass transition temperature T g , the structural relaxation time τ of a supercooled liquid rises dramatically in a narrow temperature range, until the liquid eventually becomes a glass at T g [3] . Very little structural changes accompany this process, which however leads to an extremely complex nonequilibrium state, featuring in irreversible processes like rejuvenation, memory and time asymmetry effects [4] , [5] , [6] , [7] , [8] . In addition, the response of the glass to a given perturbation, like a temperature change, strongly depends on the composition of the system and on its previous thermal history [4] , [5] , [6] , [7] , [8] , [9] . While important progress has been made in the understanding of the dynamics of glass-forming liquids [10] , [11] , [12] , [13] , a microscopic theory of glasses is still missing due to the extreme difficulty of probing the structural relaxation of a glass far below T g , either with experiments or simulations [13] , [14] , [15] , [16] , [17] . Thanks to the instrumental developments in the collection of sparse scattering signals [18] and to an increased flux and coherence of X-ray beams, X-ray photon correlation spectroscopy (XPCS) has recently emerged as a very powerful technique able to follow the evolution of the dynamics at the atomic length scale in crystalline [19] and amorphous materials [8] , [20] , [21] , [22] . Recent measurements on metallic glasses have revealed the existence of structural rearrangements at the atomic level, contrary to the common expectation of an almost arrested dynamics [8] , [20] , [21] . In those systems, the dynamics evolves from a diffusive atomic motion in the supercooled liquid, to a stress-dominated dynamics in the glass, characterized by a complex hierarchy of aging regimes. These findings present remarkable similarities with the dynamics of various complex soft materials, suggesting a more universal behaviour [23] . Among structural glasses, metallic glasses have, however, the simplest atomic structure, which is often compared with that of concentrated hard-sphere colloidal suspensions [24] . Their dynamics could therefore be not representative of the whole glassy family. Among prototypical network glasses, sodium silicates are intensively studied mainly due to their central role in geoscience and glass technology [25] , [26] , [27] , [28] , [29] . On increasing the sodium concentration, the three-dimensional network of SiO 4 tetrahedra is progressively ‘depolymerized’ by the appearance of non-bridging oxygens compensating the nearby incorporated sodium ions [25] . This process leads to a softening of the glassy matrix and significantly lowers T g [25] , [26] . On increasing the sodium concentration, the structure evolves from ‘stressed-rigid’ with independent soda-rich clusters, to a ‘floppy’ phase, characterized by interconnected soda-rich structures [26] . In this study, we elucidate the nature of the dynamics in structural glasses by monitoring the evolution of the structural relaxation time in a sodium silicate (NS4: 80%SiO 2 –20%Na 2 O), at both the atomic and mesoscopic length scales. Within the topological approach, NS4 ( T g ≈749 K) [30] lies in the intermediate stress-free glassy phase [26] . Two main features characterize its static structure factor S ( Q ): a prepeak at a wave vector Q 1 ~0.9 Å −1 , corresponding to the characteristic length scale between the sodium diffusion channels, and a dominant broad first sharp diffraction peak at Q max ~1.5 Å −1 , related to the silicon–oxygen network [27] , [28] , [31] . By exploiting the unique capabilities of XPCS, we measured the relaxation dynamics in four different NS4 glasses by performing isothermal steps in the 297–762 K temperature range, and as a function of aging, cooling rate, thermal history and wave vectors around Q 1 and Q max . Details of the different protocols are reported in the Methods section. We show that contrary to the common idea of an almost arrested dynamics, structural glasses are able to relax and rearrange their structure on a length scale of a few Angstroms. On cooling the system in the glassy state, the structural relaxation time strongly departs from the supercooled liquid behaviour and displays a weak temperature dependence, with the absence of any detectable aging not even in the glass transition region, in disagreement with macroscopic studies and theoretical approaches [4] , [5] , [6] , [7] , [15] , [29] , [32] , [33] , [34] , [35] . The relaxation time is found to be surprisingly fast, ~100–1,000 s, even hundreds of degrees below T g , in contrasts with the general idea of an ultraslow dynamics in the deep glassy state. The atomic dynamics is furthermore strongly affected by the structure and presents a peculiar slowing down at the mesoscopic length scale in correspondence to the prepeak associated with the sodium diffusion. These findings suggest the existence of a distinct relaxation dynamics at the atomic level in glasses, not taken into account by any previous study. 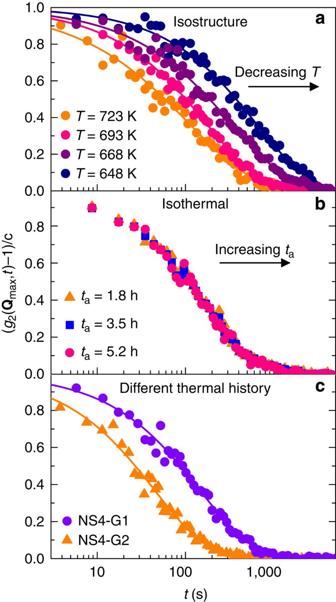Figure 1: Isostructure, isothermal and history dependence of the relaxation dynamics. Normalized intensity auto-correlation functions measured at a wave vectorQ=1.53 Å−1by means of XPCS: (a) temperature dependence of the dynamics in NS4-G1 on cooling from the supercooled liquid phase. (b) Annealing time,ta, dependence of the dynamics in NS4-G1 atT=698 K (T/Tg=0.93). (c) Intensity auto-correlation functions measured in NS4-G1 and NS4-G2 atT=713 K on cooling from the supercooled liquid phase following different thermal histories (see Methods for details). In all figures, the lines are the best fits using a Kohlrausch–Williams–Watts model function. Isostructure and history dependence study Figure 1a shows a selection of normalized temporal intensity auto-correlation functions [36] g 2 ( Q max , t ) of the NS4-G1 glass, obtained by cooling the ultraviscous melt by performing different isothermal steps. The temperature T was changed with a rate R =0.1 K min −1 in the supercooled liquid, and then with R =0.5 K min −1 in the glass. On decreasing T , the decay of g 2 ( Q max , t )−1 shifts towards longer time scales, indicating a slowing down of the atomic motion, while always displaying a full decorrelation to zero. The latter is a clear signature of an ergodic behaviour of the system at the explored atomic scale. The measured correlation functions are indeed related to the decay of the density fluctuations through the Siegert relation g 2 ( Q , t )=1+ γ | f ( Q , t )| 2 , where γ is the experimental contrast and f ( Q , t ) the intermediate scattering function [36] . It is important to stress that XPCS measures the contribution from all atoms in the scattering volume weighted by the corresponding scattering cross-sections. The presence of a frozen—thus non relaxing—component would correspond to the absence of a full decorrelation, which is not observed here. An apparent complete decay could instead arise from an incorrect sample averaging of the signal, with the consequent failure of the equivalence between the time and ensemble averaging required by the Siegert relation [37] . We ruled out this hypothesis by averaging the measured signal over the entire area of the detector and comparing the results obtained with two different detectors and on different glasses. Figure 1: Isostructure, isothermal and history dependence of the relaxation dynamics. Normalized intensity auto-correlation functions measured at a wave vector Q =1.53 Å −1 by means of XPCS: ( a ) temperature dependence of the dynamics in NS4-G1 on cooling from the supercooled liquid phase. ( b ) Annealing time, t a , dependence of the dynamics in NS4-G1 at T =698 K ( T / T g =0.93). ( c ) Intensity auto-correlation functions measured in NS4-G1 and NS4-G2 at T =713 K on cooling from the supercooled liquid phase following different thermal histories (see Methods for details). In all figures, the lines are the best fits using a Kohlrausch–Williams–Watts model function. Full size image The XPCS data are modelled with the Kohlrausch–Williams–Watts (KWW) expression g 2 ( Q max , t )−1= c *exp(−2( t / τ ) β ), where c = γ * f q 2 is the product between the contrast and the square of the nonergodicity factor f q , β is the shape parameter and τ is the relaxation time [36] . At all T , the correlation functions decay in a stretched exponential fashion with an almost constant β ~0.69±0.06, a value in agreement but slightly larger than the supercooled liquid value reported in literature ( β liquid ( T g )=0.63 (ref. 30 )). This increase could be attributed to a different relaxation mechanism in the glassy state or to a narrowing of the distribution of relaxations, which gives rise to the well-known stretched exponential behaviour observed in supercooled liquids [1] , [2] , [38] . Similar behaviour of the density fluctuations has been also reported in molecular dynamic simulations [39] , [40] and dielectric spectroscopy studies of polymeric glasses [41] . Differently from previous studies and from macroscopic measurements [4] , [5] , [6] , [7] , [15] , [29] , [32] , [33] , [34] , [35] , we do not find any evidence of physical aging on our experimental time scale of about ~4–6 h at any T , not even close to T g . While the absence of physical aging at very low temperatures has been already reported for polymeric glasses [42] , the observed stationary dynamics in the glass transition region is completely unexpected. As shown in Fig. 1b , the relaxation dynamics measured at T =698 K ( T / T g =0.93) remains stationary with τ ~300 s, even after ~10 4 s, thus waiting for a time ~70 times longer than the observed relaxation time τ . These findings are also remarkably different from the correlation functions recently observed in metallic glasses at the atomic scale [8] , [20] , [21] , since these are characterized by a fast aging and a compressed shape, thus described by β >1. In those systems, the dynamics has been attributed to the presence of internal stresses or excess free volume stored in the glass during the quenching, as in the case of many complex out-of-equilibrium soft materials [23] . In this scenario, the stretched exponential behaviour observed in NS4 might be related to its stress-free nature, as discussed in topological approaches to the glassy network [25] , [26] . A similar compressed/stressed and stretched/stress-free scenario has been recently proposed for a colloidal suspension of Laponite under an external shear field [43] . Finally, it is worth noticing that the very same absence of visible physical aging at the microscopic scale has been also detected after long annealing in metallic glasses [20] , [21] . As in those systems, the observed stationary dynamics in our silicate glasses does not correspond to an equilibrium configuration, like in supercooled liquids. Indeed, different thermal paths, or cooling rates, lead to different glassy states. This is shown in Fig. 1c where we compare the correlation functions measured at T =713 K in NS4-G1 and in a second glass, NS4-G2, obtained by cooling down the supercooled liquid with a faster rate of 1 K min −1 , leading to a faster decorrelation of g 2 ( Q max , t ). Temperature dependence of the structural relaxation time The relaxation times corresponding to NS4-G1 and NS4-G2 are shown in Fig. 2a (coloured symbols), together with relaxation times extracted from loss shear modulus experiments in the supercooled liquid at equilibrium [44] (black symbols). Both sets of XPCS data show a marked departure from the supercooled liquid at temperatures, T 1 ~742 K for NS4-G1 and T 2 ~752 K for NS4-G2, consequence of their different thermal history [4] , [45] . Albeit the different isostructures, the two glasses display a similar weak T dependence, which can be described by an Arrhenius behaviour with an extremely low activation energy of E G1 =(80±6) kJ mol −1 and E G2 =(67±8) kJ mol −1 . 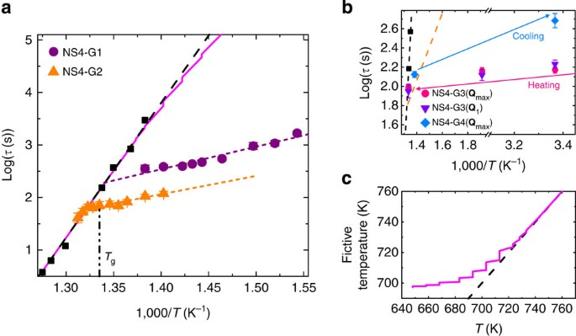Figure 2: Temperature and thermal history dependence of the structural relaxation time. (a) Arrhenius plot of the relaxation times measured with XPCS atQmax=1.53 Å−1(coloured symbols) by cooling from the ultraviscous liquid with different thermal protocols in NS4-G1 and NS4-G2 (purple circles and orange triangles, respectively). Black symbols are macroscopic data taken from the frequency dependence of the loss modulus44. The dashed lines are Arrhenius fits, while the full line is the prediction of the TNM model as explained in the text. The dash-dotted line represents the calorimetricTg=749 K30. (b) Same macroscopic data as inatogether with data taken in NS4-G3 (down triangles and circles) on heating an as-quenched glass from the room-temperature deep glassy state (at bothQ1andQmax), and in NS4-G4 (diamonds) on slowly cooling a glass that was pre-annealed 1 week at 723 K. The dashed orange line is the same as in panelaand indicates the temperature dependence in NS4-G2. Note the break in the temperature axis. (c) Fictive temperature (magenta line) as a function of the temperature estimated from the TNM model by using the thermal protocol of NS4-G1. The black dashed line is the temperature. Figure 2: Temperature and thermal history dependence of the structural relaxation time. ( a ) Arrhenius plot of the relaxation times measured with XPCS at Q max =1.53 Å −1 (coloured symbols) by cooling from the ultraviscous liquid with different thermal protocols in NS4-G1 and NS4-G2 (purple circles and orange triangles, respectively). Black symbols are macroscopic data taken from the frequency dependence of the loss modulus [44] . The dashed lines are Arrhenius fits, while the full line is the prediction of the TNM model as explained in the text. The dash-dotted line represents the calorimetric T g =749 K [30] . ( b ) Same macroscopic data as in a together with data taken in NS4-G3 (down triangles and circles) on heating an as-quenched glass from the room-temperature deep glassy state (at both Q 1 and Q max ), and in NS4-G4 (diamonds) on slowly cooling a glass that was pre-annealed 1 week at 723 K. The dashed orange line is the same as in panel a and indicates the temperature dependence in NS4-G2. Note the break in the temperature axis. ( c ) Fictive temperature (magenta line) as a function of the temperature estimated from the TNM model by using the thermal protocol of NS4-G1. The black dashed line is the temperature. Full size image At temperatures T higher than T 2 , NS4-G2 is in the supercooled liquid phase, and the corresponding relaxation times strongly vary with T , overlapping the macroscopic equilibrium values. A similar liquid-glass crossover has been also reported in metallic glasses, confirming the equilibrium restoring above T g [20] . The relatively fast dynamics and the weak T dependence reported in Fig. 2a suggest the existence of even faster atomic motion for higher cooling rates at low temperature. To check this hypothesis, we measured the atomic dynamics in another sample, NS4-G3, produced with a fast quench from the high temperature melt ( R ~100 K s −1 ) and measured at ambient temperature after ~2 years from its preparation ( Fig. 2b ). Differently from the common idea of a frozen, ultraslow dynamics, we find a relaxation time τ ~150 s at room temperature—that is, ~500 degrees below T g . This surprising fast dynamics is furthermore accompanied by an almost flat temperature dependence on heating the glass with a rate of 7 K min −1 up to T g . Interestingly, this low T dynamics remains fast even after pre-annealing a quenched glass 1 week close to T g . This is the case for NS4-G4 shown in the same figure. After the thermal treatment, the dynamics slightly slows down, signature of a very weak physical aging. Cooling this glass back to ambient T with a slow rate of 1 K min −1 , τ becomes slower than that of the pristine NS4-G3 glass with τ ~500 s, but seven orders of magnitude faster than expected from an extrapolation at low T of the NS4-G2 data obtained with the same cooling rate (dashed line). This huge difference in the microscopic relaxation times is a consequence of the strong thermal history dependence of the dynamics. NS4-G2 experiences a slow cooling across T g ( Fig. 2a ), thus after having rejuvenated the original fast quenched material. Differently, NS4-G4 keeps the memory of the fast quench and even after a thermal treatment below T g , it remains close to its original configuration. From the potential and free energy landscape approaches, the different behaviours would correspond to the existence of high energy configurational states, reachable with fast cooling rates, where the system remains trapped in a liquid-like microscopic state without having enough energy to jump into different configurations [32] , [46] , [47] , [48] . Following the Tool–Narayanaswamy–Moynihan model (TNM) [38] , [49] , [50] , [51] , we can use the thermal protocol followed during the experiments to estimate the evolution of the fictive temperature [45] and of the relaxation time that one would expect from macroscopic measurements, through the relations: with Here, is the cooling rate, T f is the fictive temperature, k B is the Boltzmann constant, t 0 is the starting point in time, x is the nonlinearity parameter and A and E a are the pre-factor and the activation energy describing the Arrhenius behaviour in the supercooled liquid phase close to T g . We numerically evaluated the model for the thermal history employed for NS4-G1 solving the above equations in a self-consistent manner starting from the equilibrium point in the supercooled liquid regime where T f = T . The parameters x =0.7 and β =0.66 are fixed to the results of calorimetric measurements reported by Moynihan et al. [52] The thermal protocol is composed of temperature changes at a constant cooling rate followed by annealing intervals of a few hours, during which the XPCS correlation functions are collected (see Methods). While the model is known to describe successfully the evolution of many macroscopic quantities in the glass transition region [49] , [50] , [51] , [52] , [53] , it fails to reproduce the XPCS data, predicting relaxation times several orders of magnitude longer than the measured ones. The model assumes indeed that the aging takes place on a time scale comparable to the structural relaxation time, and this is usually the case for macroscopic observables. Other models as well as more recent versions of the TNM one are based on the same assumption [34] , [49] , [54] , [55] . For this reason, the predicted fictive temperature ( Fig. 2c ) deviates from the actual temperature at ~714 K, where the equilibrium macroscopic relaxation time is close to the experimental time. The model thus predicts the system to have time to equilibrate during the annealing intervals even ~35 K below the calorimetric T g , according to the thermal protocol that we followed. The failure of the model to describe the XPCS relaxation time is a consequence of the absence of physical aging at the atomic level and underlines the difference with the dynamics usually observed at larger length scales. The activation energies describing the T dependence of the atomic dynamics shown in Fig. 2a are very close to that reported in literature for the sodium diffusion. The latter however corresponds to relaxation times many orders of magnitude faster than those observed here [56] , [57] , [58] . This is shown in Fig. 3 comparing the Na and Si–O diffusion constants with the effective diffusion coefficients extracted from the XPCS relaxation times of NS4-G2 and NS4-G3. The latter has been calculated through the relation D xpcs =1/( τ incoh Q 2 ), being the incoherent contribution to the relaxation time given by τ incoh = τ xpcs / S ( Q ) [59] . The dynamics measured with XPCS is more than 10 orders of magnitude slower than that of sodium diffusion, while it is clearly closer to the low T extrapolation of the Si–O matrix dynamics. 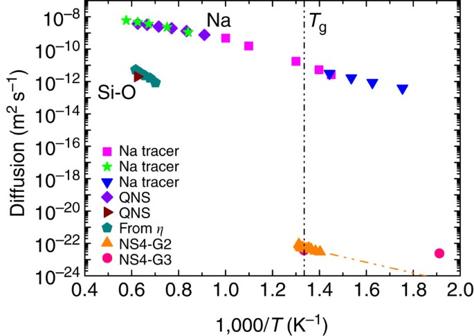Figure 3: Comparison with diffusion data. Sodium and Si–O diffusion data taken from Na tracers, quasi elastic neutron scattering (QNS) and viscosityη56,57, together with the effective diffusion coefficientDxpcsestimated from the XPCS relaxation times in NS4-G2 and NS4-G3. The dot-dashed orange line describes the Arrhenius temperature dependence of NS4-G2 in the glassy state, while the black vertical line corresponds to the calorimetric glass transition temperature30. Figure 3: Comparison with diffusion data. Sodium and Si–O diffusion data taken from Na tracers, quasi elastic neutron scattering (QNS) and viscosity η [56] , [57] , together with the effective diffusion coefficient D xpcs estimated from the XPCS relaxation times in NS4-G2 and NS4-G3. The dot-dashed orange line describes the Arrhenius temperature dependence of NS4-G2 in the glassy state, while the black vertical line corresponds to the calorimetric glass transition temperature [30] . Full size image Wave vector dependence study Albeit the large difference in diffusion constants, the atomic dynamics is strongly affected by the presence of sodium in the glassy matrix, resulting in a peculiar wave vector dependence of the relaxation time at the mesoscopic scale. This is shown in Fig. 4a where we report the low T behaviour of τ ( Q ) and S ( Q ) in NS4-G3. While S ( Q ) presents a unique broad maximum at the tetrahedral distance, the relaxation time exhibits a distinct Q dependence, characterized by a broad peak with two contributions: a maximum value at Q 1 ~0.9 Å −1 and a pronounced shoulder close to Q max ~1.53 Å −1 , the latter being close to the first maximum of the S ( Q ). Interestingly, Q 1 corresponds to the well-known prepeak attributed to the preferential ion-conducting pathways in the structure of sodium silicate glasses [27] , which appears only as a very tiny shoulder in the static data. A very similar behaviour, with τ ( Q 1 )~ τ ( Q max ), has indeed been observed in molecular dynamics simulations of molten sodium silicates [28] , [31] , but it has never been seen experimentally. Our data not only confirm this remarkable structural influence on the dynamics, but also show that it persists even in the deep glassy state, and presents the same weak temperature dependence than τ ( Q max ) (see Fig. 2b for a comparison between τ ( Q max , T ) and τ ( Q 1 , T )). 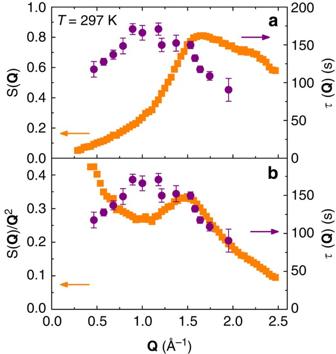Figure 4: Wave vector dependence of the relaxation time. (a) Relaxation times measured in the ‘as-quenched glass’ NS4-G3 for different wave vectorsQ(circles) together with the corresponding static structure factor (squares). (b) Sameτ(Q) data together with theS(Q) rescaled byQ2. Figure 4: Wave vector dependence of the relaxation time. ( a ) Relaxation times measured in the ‘as-quenched glass’ NS4-G3 for different wave vectors Q (circles) together with the corresponding static structure factor (squares). ( b ) Same τ ( Q ) data together with the S ( Q ) rescaled by Q 2 . Full size image On the other hand, the shoulder around Q max is reminiscent of the de Gennes-like narrowing observed in coherent neutron scattering experiments of supercooled liquids [60] , [61] , [62] , [63] . This feature is better evidenced by comparing τ ( Q ) with the quantity S ( Q )/ Q 2 as shown in Fig. 4b . Albeit the clear disagreement at low Q s, the two quantities agree quite well for wave vectors larger than 1.3 Å −1 . At lower Q s, the relaxation time is dominated by the additional contribution to the dynamics related to the sodium diffusion channels in the matrix and deviates from the de Gennes picture. This peculiar behaviour of τ ( Q ) persists on temperature increase (see Fig. 2b and Fig. 5 ) and strongly resembles that reported in few coherent neutron scattering studies of polymeric supercooled liquids [61] , [62] , [63] . In these systems, the dynamics is affected by two main contributions, which lead to an oscillatory behaviour of τ ( Q ) with a first maximum in correspondence with a weak structural prepeak, followed by a second one associated with the de Gennes narrowing at the main sharp diffraction peak. As in the case of silicates, the relaxation time displays a similar value at the wave vectors corresponding to the two structural features but in the very fast time domain of ~10 −9 s, thus for relaxation times 12 orders of magnitude faster than those probed here by XPCS. The particular Q dependence of τ in supercooled liquids has been recently attributed to the decoupling between diffusion and viscosity and a growing dynamic length scale [64] , [65] . 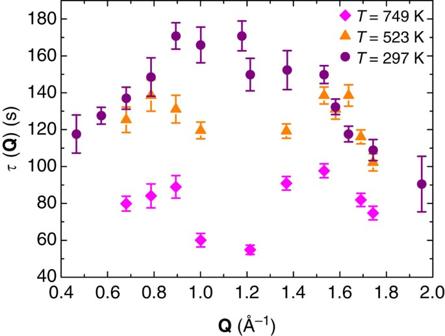Figure 5: Temperature evolution of the wave vector dependence of the relaxation time. Evolution of the wave vector dependence of the relaxation time measured in NS4-G3 on heating the system from 297 K up to the calorimetricTg. Figure 5: Temperature evolution of the wave vector dependence of the relaxation time. Evolution of the wave vector dependence of the relaxation time measured in NS4-G3 on heating the system from 297 K up to the calorimetric T g . Full size image We have presented the first measurements that follow the time and temperature evolution of the density fluctuations in a network glass at both the mesoscopic and atomic length scales. Our study reveals the existence of fast collective atomic motion in the glassy state, in contradiction with the common idea of an almost arrested out-of-equilibrium state. Differently from macroscopic studies, the relaxation dynamics remains stationary even in the glass transition region; thus, for temperatures where the annealing time is much longer than the structural relaxation time, one would expect from a simple extrapolation starting from supercooled liquid relaxation times. These results indicate a different physical mechanism responsible for the relaxation dynamics at the microscopic level unaccounted for in previous experimental and theoretical works. Our findings suggest indeed the existence of microscopic liquid-like dynamical regions, surrounded by a macroscopically nonrelaxing structure, whose motion strongly depends on the previous thermal history of the sample. From the energy landscape point of view [32] , [45] , [46] , [47] , this description would correspond to the existence of different sub-minima of similar energy barriers that the system can explore with relaxation times of the order of 100–1,000 s. The experimental detection of such local atomic motion in the macroscopically large scattering volume suggests the existence of many different independent groups of atoms, which move rapidly among the sub-minima of a deep local minimum. Albeit a similar description has been often associated with secondary relaxation processes active in the glassy state [1] , [53] , [66] , [67] , [68] , we ruled out this hypothesis because in this case the correlation curves would decay towards a long nonergodic plateau, indicating the existence of a much slower final decay associated with the structural relaxation process. Differently, our data display a full decorrelation to zero of the density fluctuations, suggesting the main structural relaxation to be responsible of the observed decorrelation at the atomic level. In addition, this decay occurs in a stretched exponential way, which can be described by a shape exponent β close to the value reported in literature for the structural relaxation process in the corresponding supercooled liquid phase. This interpretation is furthermore supported by the fact that the measured relaxation times match with macroscopic structural relaxation times at the glass transition temperature and in the supercooled liquid phase. The microscopic relaxation dynamics is in addition significantly affected by the presence of ion-conducting pathways, presenting a peculiar increase in the relaxation time at the characteristic distance between the sodium diffusion channels in the network, in agreement with high temperature simulation in molten silicates [28] , [31] . A similar Q dependence has been reported also in few other supercooled liquids, but for very high temperatures and for time scales more than 10 orders of magnitude faster than those here probed [62] , [63] , suggesting a more complex origin [64] , [65] . The existence of structural rearrangements for temperatures far below T g has been recently reported by applying external stimuli [16] and in macroscopic studies [17] . In this latter case, the authors attributed the macroscopic strain relaxation of the glass to the presence of mixed alkali ions in the network [17] . Our results in a single-alkali glass broaden and strengthen the results reported in ref. 17 by showing the first direct experimental evidence of the spontaneous atomic motion in glasses, and they therefore keep the promise to significantly improve our knowledge of disordered systems. The relaxation dynamics of silicate glasses strongly differ from that recently reported for metallic glasses [8] , [20] , [21] . In these systems, the atomic motion appeared to be governed by the presence of internal stresses stored in the system during the quenching, suggesting a ballistic nature of the dynamics as in the case of many complex soft materials [23] , [69] . These internal stresses are then partially released on increasing the temperature, leading to distinct aging regimes. Differences in the atomic mobility and in the microscopic elasticity are likely to be the reason of the observed behaviours. However, whether this is a universal difference between metallic and network glasses requires further investigation. Finally, it is worth emphasizing that this kind of microscopic studies will strongly benefit from the future upgrade of the storage ring facilities and from the advent of the free electron lasers sources, opening the field to a wide range of investigations. Materials and thermal protocols Samples of 0.8 SiO 2 –0.2 Na 2 O glass were prepared by melting pure SiO 2 and Na 2 CO 3 at 1,870 K in air in an alumina crucible for several hours. The melt was quenched below T g by immersion of the crucible in water, resulting in a quenching rate of the order of 100 K s −1 . Transparent cylindrical samples were extracted from the crucible using a diamond milling head of 5 mm diameter. The optimal thickness of the sample was chosen to optimize the scattered intensity at 8 keV while keeping a reasonably good contrast. For this reason, ~50-μm-thick glasses were used for the experiments, resulting in an experimental contrast of ~2% and a sample transmission of ~66%. A resistively heated furnace in Ni was used for the measurements. The samples were mounted on a specifically designed sample holder with an internal cylindrical shape (5 mm external diameter with a 2-mm hole in the middle for the X-rays). The temperature was measured by a thermocouple inserted close to the sample and was monitored during the whole experiment. The temperature stability was 0.1 K. NS4-G1 : The sample was first annealed above T g at 783 K and then slowly cooled down to 723 K through different isothermal steps with a rate of 0.1 K min −1 between the steps in a total period of 22 h. This protocol was chosen to allow the system to follow the temperature changes in the highly viscous supercooled liquid region. XPCS measurements were performed on cooling the system in the 723–648 K temperature range with a rate of 0.5 K min −1 and by performing isothermal steps of ~4–6 h at each temperature. NS4-G2 : The sample was first annealed above T g at 775 K and then slowly cooled down to 762 K with a rate of 1 K min −1 . The isothermal XPCS measurements were performed on cooling the system in the 762 K–713 K temperature range with a rate of 1 K min −1 and staying ~1.3 h at each temperature. NS4-G3 : The sample was prepared by a fast quenching ( R ~100 K s −1 ) from the high temperature melt and kept at ambient temperature (297 K) for ~1.5 years in the laboratory. After measuring at room temperature, the sample was heated up to 523 and 749 K with a rate of 7 K min −1 , by performing isothermal steps of ~20 h at each temperature. NS4-G4 : Fast-quenched sample (as NS4-G3)was first annealed below T g at 723 K for 1 week and then cooled down to 297 K. The temperature was changed with a heating and cooling rate of 3 and 1 K min −1 , respectively. X-ray photon correlation spectroscopy XPCS measurements were performed at the beamline ID10 at the ESRF. An X-ray beam, produced by an undulator source, was focused by a Be compound refractive lens and 8 keV radiation was selected by a Si(111) monochromator reflection (energy bandwidth Δ E / E =1.4 × 10 −4 ). Higher harmonics were suppressed by two Si mirrors reflecting at a grazing incident angle of 0.2°. A partially coherent beam was selected by rollerblade slits opened to 10 × 10 μm 2 , placed ~0.18 m upstream of the sample, providing a flux of ~10 10 –10 11 photons per second per 200 mA, depending on the experiment. This configuration results in a longitudinal coherence length of ~1.1 μm and a transverse coherence length of ~4 μm (H) × 10 μm (V). To enhance the total measured signal, speckle patterns were recorded by using two IkonM charge-coupled devices (CCD) from Andor Technology (1024 × 1024 pixels, 13 × 13 μm 2 pixel size) installed perpendicularly to the horizontal scattering plane, ~67 cm downstream of the sample, and symmetrically with respect to the incoming beam. In this way, the two detectors cover the same solid angle and the same wave vector Q with a resolution of ΔQ =0.04 Å −1 . The scattered intensity was collected in the horizontal plane for wave vector Q between 0.3–2.0 Å −1 and for different temperatures in the 297–762 K range. At each temperature series up to 4,000 frames with 3, 5 and 7 s, exposure time per frame were collected. The data were treated and analysed following the procedure described in ref. 18 to calculate the temporal intensity auto-correlation functions where I p ( Q , t 1 ) and I p ( Q , t 1 + t ) correspond to the intensity measured on the pixel p at the time t 1 and t 1 + t , <…> p is the ensemble average over all the pixels of the detector, which correspond to the same wave vector Q , and <...> t 1 is the temporal average over all times t 1 . In the wide angle configuration here employed, all pixels of the CCD were considered to belong to the same Q . To investigate the presence of physical aging, we compared sets of ~1,000 frames measured at different annealing times. The latter quantity was defined as t a = t 0 +( t f − t i )/2, being t 0 the elapsed time from temperature equilibration and the beginning of the used sets of images, and t f and t i the final and starting time of the set, respectively. As explained in refs 20 and 21 , XPCS allows studying the physical aging in glasses because the time necessary for a measurement is shorter than the aging time of the sample. The amorphous structure of the sample was checked before and after each acquisition by measuring the intensity I ( Q ) in the 0.4–2.5 Å −1 Q range. The S ( Q ) has been determined from the measured intensity using an SiO 2 sample as a reference and taking into account the Q dependence of the atomic form factors and the effect of the linear polarization of the X-ray beam in the horizontal plane. Three synchrotron experiments of 1 week each have been performed to measure the whole set of data, while the reproducibility of the results was checked by using different glasses and measuring at distinct sample positions. To control the absence of any systematic changes during the measurements, the Q dependence of the relaxation time measured at ambient temperature ( T =297 K) in NS4-G3 was obtained by collecting images at different sample positions for each Q , and low and high Q values were measured in an alternate way. The reproducibility of the data was also checked by repeating the data acquisition at some selected Q s (see Fig. 6 ). 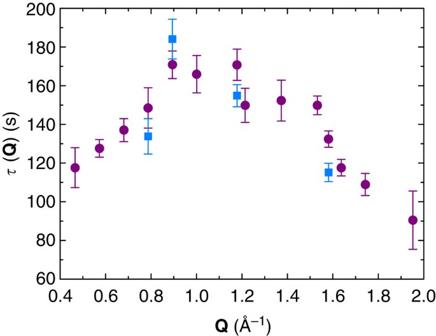Figure 6: Reproducibility of the wave vector dependence of the relaxation time. Wave vector dependence of the relaxation time measured at 297 K in NS4-G3 (circles). The dynamics at some selectedQs was measured two times (squares) to check the reproducibility of the data. Figure 6: Reproducibility of the wave vector dependence of the relaxation time. Wave vector dependence of the relaxation time measured at 297 K in NS4-G3 (circles). The dynamics at some selected Q s was measured two times (squares) to check the reproducibility of the data. Full size image The stability of the technique was furthermore checked by monitoring the intensity after the beam defining slits and by measuring the dynamics in a reference sample, a Pd-based metallic glass, which has relaxation times of more than 10 4 s, with a long initial nonergodic plateau up to ~1,500 s (see Fig. 7 ). This measurement was performed by using exactly the same experimental setup as for the silicate glasses and it has been used as reference for the experimental contrast (which is ~5% in this glass) and the stability of the technique. As shown in the figure, the dynamics of the system is extremely slow and the correlation function displays a long nonergodic plateau up to ~1,500 s, after which it starts to decay in a compressed exponential way, in agreement with the results on other metallic glasses [8] , [20] , [21] . 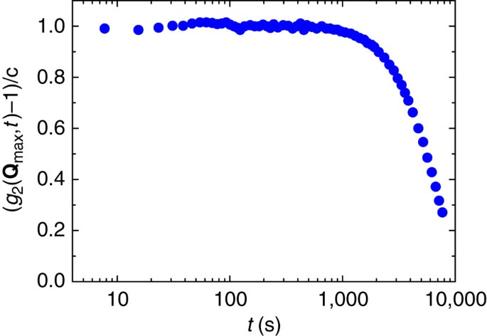Figure 7: Mechanical stability of the experimental setup. Intensity correlation function measured with XPCS in a Pd77Si16.5Cu6.5metallic glass at 323 K and forQ=2.5 Å−1. The measurement was performed during the experiment on silicate glasses and by using the same setup. Figure 7: Mechanical stability of the experimental setup. Intensity correlation function measured with XPCS in a Pd 77 Si 16.5 Cu 6.5 metallic glass at 323 K and for Q =2.5 Å −1 . The measurement was performed during the experiment on silicate glasses and by using the same setup. Full size image The relaxation dynamics measured in our silicate glasses cannot be induced neither by any artificial drifts of the illuminated sample position. We performed numerical simulations showing that the sample should move by ~60% of the beam size (Gaussian shape) to reduce ( g 2 ( Q max, t )–1)/ c by a factor equal to e −1 . This would correspond to a shift of ~6 μm of the illuminated sample position, a value which is incompatible with the stability of both the sample position and the incoming X-ray beam. The furnace is mounted on a massive Huber stage with motors having a precision of ~0.1 μm. On the other hand, the X-ray beam produced at ESRF has submicron stability and the intensity after the 10 × 10 μm 2 aperture of the beam defining slits has been always controlled by a monitor placed between the slits and the sample. Finally, it is worth mentioning that a drift in the scattering volume would lead to a compressed exponential decay of the correlation functions with a shape parameter β ~2 in disagreement with the stretched exponential decay observed in our silicate glasses. How to cite this article: Ruta, B. et al. Revealing the fast atomic motion of network glasses. Nat. Commun. 5:3939 doi: 10.1038/ncomms4939 (2014).